Stable Li-ion battery anodes byin-situpolymerization of conducting hydrogel to conformally coat silicon nanoparticles Silicon has a high-specific capacity as an anode material for Li-ion batteries, and much research has been focused on overcoming the poor cycling stability issue associated with its large volume changes during charging and discharging processes, mostly through nanostructured material design. Here we report incorporation of a conducting polymer hydrogel into Si-based anodes: the hydrogel is polymerized in-situ , resulting in a well-connected three-dimensional network structure consisting of Si nanoparticles conformally coated by the conducting polymer. Such a hierarchical hydrogel framework combines multiple advantageous features, including a continuous electrically conductive polyaniline network, binding with the Si surface through either the crosslinker hydrogen bonding with phytic acid or electrostatic interaction with the positively charged polymer, and porous space for volume expansion of Si particles. With this anode, we demonstrate a cycle life of 5,000 cycles with over 90% capacity retention at current density of 6.0 A g −1 . Developing rechargeable lithium-ion batteries with high-energy density and long cycle life is of critical importance to address the ever-increasing energy storage needs for various technological applications, including portable electronics, hybrid and electric vehicles, and grid-scale energy storage systems [1] , [2] , [3] , [4] . Graphite, the traditional anode material in lithium-ion batteries does not meet with high energy needs due to its limited theoretical specific capacity of ~370 mAh g −1 . Silicon (Si) has attracted a great deal of attention as an alternative anode material for Li-ion batteries lately [5] , [6] , [7] , [8] , primarily due to: (1) its high theoretical gravimetric capacity of ~4,200 mAh g −1 based on the Si weight, (2) its relatively low discharge potential (~0.5 V versus Li/Li + ), (3) the natural abundance of elemental Si, and (4) its safety and environmental benignity [9] , [10] , [11] , [12] , [13] , [14] , [15] , [16] , [17] . However, Si-based anodes also face significant challenges due to the ~400% volume expansion upon lithium insertion in Si [18] ; this can result in fracture and loss of electrical contact, and an unstable solid electrolyte interphase (SEI) growth on the Si surface [19] . Recently, exciting progress has been made through nanostructuring of Si. Nanocrystals [20] , nanowires [21] , core-shell nanofibers [22] , [23] , nanotubes [16] , nanospheres [24] , nanoporous materials [25] and Si/carbon nanocomposites [26] , [27] have all shown longer cycling life as candidate anode materials compared with micron-sized Si particles [12] , [13] , [16] , [21] , [22] , [25] , [26] , [27] . In addition, fundamental studies using in-situ X-ray, electron microscopy, and mechanical modelling have helped elucidate the nature of Li–Si reactions [6] , [7] , [8] , [28] , [29] . However, synthesis of Si nanostructures usually involves high temperature chemical vapour deposition or complex chemical reactions and/or templates, [11] , [21] , [22] , [23] , [24] , [25] and their scalability and compatibility with existing battery manufacturing processes remain a challenge. More recently, electrodes made from Si nanoparticle (SiNP) slurries have been investigated by several research groups as a potentially manufacturing-compatible route [25] , [26] , [30] , [31] . Various polymer binders other than traditional polyvinylidene difluoride (PVDF), including polyacrylic acid (PAA), carboxy-methyl cellulose (CMC), poly(9,9-dioctylfluorene-co-Suorenone-co-methylbenzoic acid) (PFFOMB) and alginate, have been found to enhance the cycle life [14] , [15] , [32] , [33] , [34] , [35] , [36] . The cycle life improvement when using PAA, CMC and alginate binders was attributed to the high polymer modulus values and the binding between the functional groups on the polymers with the surface oxide on the Si particles. In the case of the PFFOMB binder, an interesting concept was demonstrated that combined binding and conducting properties in the binder molecules [5] . Building on the previous work on polymer binders, here we demonstrate that a unique feature of our approach for realizing this excellent performance is the use of in-situ polymerization, to form a bi-functional conformal coating that binds to the Si surface and also serves as a continuous three-dimensional (3D) pathway for electronic conduction. The in-situ polymerization fabrication technique is quite different from previous studies, where the direct mixing of Si particles with polymer binders produces less conformal coatings and non-continuous electronic transport pathway. Material and structural design Conductive polymer hydrogels are unique materials that offer advantages such as a 3D hierarchical porous-conducting framework and excellent electronic and electrochemical properties [37] . Recently, we have shown that they exhibit superior electrochemical performance when used in supercapacitors and ultrasensitive biosensors [38] . The 3D porous micro- and nanostructures of conductive polymer hydrogels can promote the transport of both electrons and ions owing to the availability of short diffusion paths and good 3D connectivity. Moreover, they can be synthesized by simply mixing two solutions, where one contains the initiator (oxidizer) and the other contains the crosslinker and the monomer. For example, phytic acid, a naturally occurring molecule consisting of six phosphoric acid groups, can be used as both the gelator and dopant to react with the aniline monomer by protonating the nitrogen groups on polyaniline (PANi), leading to the formation of a 3D interconnected network structure [38] . In this work, when SiNPs are mixed into the solution during polymerization, the phosphoric acid groups in the phytic acid molecules can potentially bind with the SiO 2 on the Si particle surfaces via hydrogen bonding, which was thought to contribute to the improved cycle lifetime for PAA, CMC and alginate binders with carboxylic acid groups [32] , [33] , [34] , [36] . This interaction can also result in the conformal coating of phytic acid molecules on the surface, which may further crosslink with aniline monomers during polymerization to generate a conformal conductive coating. Additionally, the negatively charged surface oxide may electrostatically interact with the positively charged PANi doped by the phytic acid [39] . All the above interactions result in the formation a 3D continuous-conducting hydrogel network, trapping the coated Si particles inside ( Fig. 1a ). 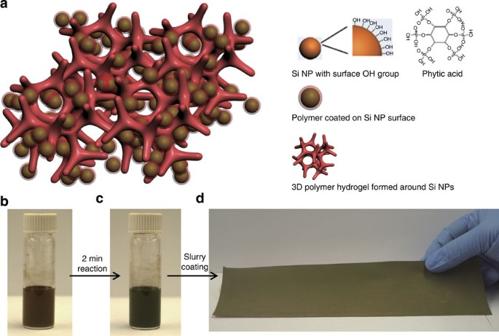Figure 1: Electrode design and fabrication. (a) Schematic illustration of 3D porous SiNP/conductive polymer hydrogel composite electrodes. Each SiNP is encapsulated within a conductive polymer surface coating and is further connected to the highly porous hydrogel framework. SiNPs has been conformally coated with a polymer layer either through interactions between surface -OH groups and the phosphonic acids in the crosslinker phytic acid molecules (right column), or the electrostatic interaction between negatively charged -OH groups and positively charge PANi due to phytic acid doping. (b–d) Photographs showing the key steps of the electrode fabrication process. (b) First, SiNPs were dispersed in the hydrogel precursor solution containing the crosslinker (phytic acid), the monomer aniline and the initiator ammonium persulphate. (c) After several minutes of chemical reaction, the aniline monomer was crosslinked, forming a viscous gel with a dark green colour. (d) The viscous gel was then bladed onto a 5 × 20 cm2copper foil current collector and dried. Figure 1: Electrode design and fabrication. ( a ) Schematic illustration of 3D porous SiNP/conductive polymer hydrogel composite electrodes. Each SiNP is encapsulated within a conductive polymer surface coating and is further connected to the highly porous hydrogel framework. SiNPs has been conformally coated with a polymer layer either through interactions between surface -OH groups and the phosphonic acids in the crosslinker phytic acid molecules (right column), or the electrostatic interaction between negatively charged -OH groups and positively charge PANi due to phytic acid doping. ( b – d ) Photographs showing the key steps of the electrode fabrication process. ( b ) First, SiNPs were dispersed in the hydrogel precursor solution containing the crosslinker (phytic acid), the monomer aniline and the initiator ammonium persulphate. ( c ) After several minutes of chemical reaction, the aniline monomer was crosslinked, forming a viscous gel with a dark green colour. ( d ) The viscous gel was then bladed onto a 5 × 20 cm 2 copper foil current collector and dried. Full size image Material synthesis and electrode fabrication The SiNP-PANi hydrogel composite is prepared via a scalable solution phase synthesis by mixing SiNPs with phytic acid and aniline in water to give a brown suspension ( Fig. 1b ). Within 3 min upon adding an oxidizer (for example, ammonium persulphate), the aniline was observed to rapidly polymerize and crosslink, resulting in a dark green viscous gel due to the presence of the phytic acid gelator ( Fig. 1c ). The viscous gel was then bladed onto a copper foil current collector and dried to form a uniform film over a large area; Fig. 1d shows an example of a uniformly coated electrode film (5 cm × 20 cm). This solution-based synthesis method and its compatibility with roll-to-roll coating methods make this system readily scaled for large area electrode films [40] . The SiNP-PANi hydrogel composite film was then thoroughly washed in deionized water to remove excess ions and oligomers, followed by vacuum drying overnight. 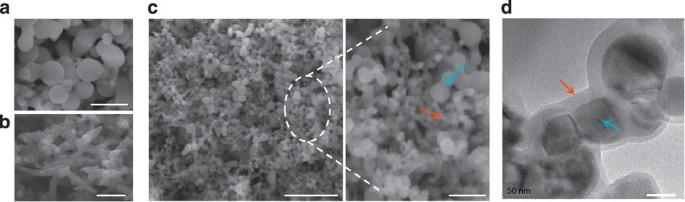Figure 2: Microstructure of the SiNP-PANi composite electrodes. (a) SEM image of pure SiNPs. Scale bar, 200 nm. (b) SEM image of the PANi hydrogel sample. Scale bar, 100 nm. (c) SEM image of a SiNP-PANi composite electrode at low (left) and high (right) magnifications. Scale bar, 1 μm (left) and 200 nm (right). The blue arrow indicates SiNPs while the red arrow shows the PANi hydrogel network. (d) A TEM image shows that the SiNPs (blue arrow) are coated with a uniform PANi polymer layer (red arrow). Scale bar, 50 nm. Figure 2 shows scanning electron microscopy (SEM) images of the SiNP-PANi hydrogel composite electrodes. Typically, the spherical silicon nanoparticles have an average diameter of ~60 nm ( Fig. 2a ), while the dried polymer hydrogel consists of a hierarchical 3D porous foam-like network composed of dendritic nanofibers with typical diameters of 60–100 nm ( Fig. 2b ). As the PANi was formed in the presence of the SiNPs, the SiNPs are in intimate contact with the conductive polymer hydrogel matrix at both the microscopic and molecular level. This is confirmed by SEM images of the composite electrode ( Fig. 2c ), which clearly show a uniform mixture of SiNPs embedded inside the highly porous polymer matrix. Additionally, SiNPs appear to be encapsulated by a conformal PANi coating due to the in-situ polymerization discussed above, as shown in the transmission electron microscopy (TEM) image ( Fig. 2d ). As will be discussed later, the superior electrochemical performance of the Si-PANi hydrogel composite electrodes can be attributed to the advantageous features offered by the unique hierarchical microstructure. Figure 2: Microstructure of the SiNP-PANi composite electrodes. ( a ) SEM image of pure SiNPs. Scale bar, 200 nm. ( b ) SEM image of the PANi hydrogel sample. Scale bar, 100 nm. ( c ) SEM image of a SiNP-PANi composite electrode at low (left) and high (right) magnifications. Scale bar, 1 μm (left) and 200 nm (right). The blue arrow indicates SiNPs while the red arrow shows the PANi hydrogel network. ( d ) A TEM image shows that the SiNPs (blue arrow) are coated with a uniform PANi polymer layer (red arrow). Scale bar, 50 nm. Full size image Electrochemical performance To characterize the electrochemical properties of SiNP-PANi composite electrodes, cyclic voltammetry (CV) measurements were performed on half cells at a scan rate of 0.1 mV s −1 over the potential window of 0.01–1 V versus Li/Li + ( Fig. 3a ). As shown in Fig. 3a , the CV profile (red curve) of a SiNP-PANi hydrogel composite electrode exhibits similar electrochemical characteristics as that of pristine Si powders [26] . The peak at 0.19 V in the cathodic process corresponds to the conversion of crystalline Si to the Li x Si phase, while the two peaks at 0.41 and 0.53 V in the anodic process correspond to the delithiation of amorphous (α) α-Li x Si to α-Si [26] . For comparison, the CV profile of a dried PANi hydrogel film (blue line in Fig. 3a ) shows that the current density is about two orders of magnitude lower than that of the composite electrode, indicating negligible contribution from PANi to the capacity of the whole electrode. 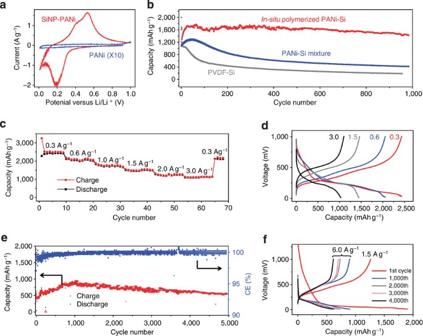Figure 3: Electrochemical characteristics. (a) CV measurement of SiNP-PANi hydrogel composite (red line) and PANi hydrogel (blue line) at a scan rate of 0.1 mV s−1over the potential window of 0.01–1 V versus Li/Li+. (b) Electrochemical cycling performance of thein-situpolymerized SiNP-PANi composite electrodes under deep charge/discharge cycles from 1 to 0.01 V with a charge/discharge current of 1.0 A g−1, showing stable capacity of ~1,200 mAh g−1after 1,000 cycles (red line). Electrochemical cycling of control samples are compared in the figure. Blue line: SiNP-PANi withoutin-situpolymerization. Green line: PVDF-SiNP electrode. (c) Capacity and (d) galvanostatic charge/discharge profiles of a SiNP-PANi electrode cycled at various current densities: 0.3, 0.6, 1.0 and 3.0 A g−1(from right to left). (e) Lithiation/delithiation capacity and CE of SiNP-PANi electrode cycled at current density of 6.0 A g−1for 5,000 cycles. (f) Galvanostatic charge/discharge profiles plotted for the 1st, 1,000th, 2,000th, 3,000th and 4,000th cycles. All electrochemical cycling measurements (b–f) were carried out at room temperature in two-electrode 2032 coin-type half-cells. All the specific capacities and current density are reported based on the weight of SiNPs. Figure 3: Electrochemical characteristics. ( a ) CV measurement of SiNP-PANi hydrogel composite (red line) and PANi hydrogel (blue line) at a scan rate of 0.1 mV s −1 over the potential window of 0.01–1 V versus Li/Li+. ( b ) Electrochemical cycling performance of the in-situ polymerized SiNP-PANi composite electrodes under deep charge/discharge cycles from 1 to 0.01 V with a charge/discharge current of 1.0 A g −1 , showing stable capacity of ~1,200 mAh g −1 after 1,000 cycles (red line). Electrochemical cycling of control samples are compared in the figure. Blue line: SiNP-PANi without in-situ polymerization. Green line: PVDF-SiNP electrode. ( c ) Capacity and ( d ) galvanostatic charge/discharge profiles of a SiNP-PANi electrode cycled at various current densities: 0.3, 0.6, 1.0 and 3.0 A g −1 (from right to left). ( e ) Lithiation/delithiation capacity and CE of SiNP-PANi electrode cycled at current density of 6.0 A g −1 for 5,000 cycles. ( f ) Galvanostatic charge/discharge profiles plotted for the 1st, 1,000th, 2,000th, 3,000th and 4,000th cycles. All electrochemical cycling measurements ( b – f ) were carried out at room temperature in two-electrode 2032 coin-type half-cells. All the specific capacities and current density are reported based on the weight of SiNPs. Full size image The electrochemical cycling performance of the composite electrodes was evaluated using deep charge/discharge galvanostatic cycling from 1 to 0.01 V ( Fig. 3b–e ). The first charge has a long plateau around 0.1 V, which corresponds to the lithiation potential of pure crystalline silicon ( Supplementary Fig. S1 ). At a charge/discharge current of 1.0 A g −1 , the SiNP-PANi composite electrode exhibits a relatively stable reversible lithium capacity of 1,600 mAh g −1 for 1,000 deep cycles based on the weight of only Si ( Fig. 3b ). In comparison, the SiNP electrode using traditional PVDF binder loses >50% of its initial capacity after being cycled only 100 times ( Fig. 3b ). The volumetric capacity of the SiNP-PANi hybrid electrode is estimated to be ~1,080 mAh cm −3 (see supporting information for calculation details), which is about double that of graphite electrode (~ 620 mAh cm −3 ) [33] , but lower than the volumetric capacity for SiNP-alginate electrode reported in Kovalenko et al . [33] (~1,520 mAh cm −3 ). This is mainly due to the 3D porous structure of the whole electrode as presented in Fig. 2c . The active Si material mass loading has an important role for practical battery applications. The Si mass loading in the present study is typically 0.2–0.3 mg cm −2 , which is similar to that of Si/PFFOMB electrode reported by Liu et al . [32] (0.3 mg cm −2 for total mass loading, and 0.2 mg cm −2 Si mass loading). We note that although this value is low for practical battery application, the mass loading can be potentially increased by multiple depositions of materials, which is an important aspect to investigate for future studies. The continuous-conducting polymer hydrogel framework, which is directly connected to the current collector, provides channels for fast electron transport, thereby enabling outstanding rate capability. As shown in Fig. 3c , the capacity of a SiNP-PANi composite electrode varies from 2,500 mAh g −1 to 1,100 mAh g −1 at charge/discharge rate from 0.3 to 3.0 A g −1 . Fig. 3d shows that even at a high charge/discharge current of 3.0 A g −1 , the lithiation potential still shows a sloping profile between 0.3 and 0.01 V, consistent with previously reported Li insertion to form amorphous Li x Si [11] . Clearly, Li + ions can rapidly pass through the thin PANi layer to reach the silicon active material even at high charge/discharge rates. To obtain long cycling results within a reasonable testing period, faster charge and discharge tests with deep cycling (1 to 0.01 V) were carried out. Figure 3e shows that at a high current density of 6.0 A g −1 , an electrode capacity of ~550 mAh g −1 was still retained after 5,000 cycles, which corresponds to ~91% capacity retention at current density of 6.0 A g −1 . No obvious changes in the charge capacity or charge/discharge profiles can be found after 5,000 cycles for the Si-PANi hybrid anode ( Fig. 3f ), indicating its superior and stable cycling performance. We note that an increase of the capacity of the in-situ polymerized PAN-Si anode was observed during the initial cycles ( Fig. 3b ). The origin of this activation step can be possibly attributed to the delayed wetting of electrolyte into the 3D nanoporous structure of the composite electrode. High coulombic efficiency (CE) is required for practical silicon-based electrodes. For our Si-PANi hydrogel composite electrodes, the CE of the first cycle was usually ~70% because SEI formation consumes a certain percentage of the lithium; this could be improved by prelithiation in future studies ( Fig. 3e ). The average CE of the composite electrode from the 2nd to 5,000th cycle is 99.8%, which is higher than that previously reported for silicon nanoparticles and nanowires [21] , [25] . The high CE achieved here is due in large part to the formation of a stable SEI on the composite electrode, which we will discuss in greater details later. We attribute the above demonstrated exceptional electrochemical stability to the unique nanoscale architecture of the Si-PANi composite electrode. First, the porous hydrogel matrix has empty space to allow for the large volume expansion of the SiNPs during lithium insertion. Second, the highly conductive and continuous 3D PANi framework, as well as the conformal conductive coating surrounding each SiNP, helps provide good electrical connection to the particles. Third, although pulverization of larger particles may still occur during lithiation and battery cycling, the fractured Si pieces are trapped within the interconnected narrow pores of the polymer matrix, maintaining good electrical connectivity among fractured particles. TEM images showed that even after 2,000 electrochemical cycles, SiNPs are still inside the polymer matrix without losing electrical contact ( Supplementary Fig. S2 ). Even though we observed that the polymer surface coating on the particles broke upon initial volume expansion during lithiation, the coating still nonetheless enabled the SiNPs to remain connected to the conductive matrix ( Supplementary Fig. S2 ). To further confirm the stabilizing effect of the in-situ polymerized PANi coating, we fabricated a control electrode by mixing pre-synthesized PANi hydrogel and SiNPs. In this control sample, a similar weight ratio of the SiNPs to the PANi hydrogel composite structure was used, but there was no intimate surface coating on the Si particles as the aniline precursor had already been polymerized before mixing. The electrochemical cycling of this control sample is presented in Fig. 3b . Even though this system showed better cycling stability than the bare SiNP electrode with PVDF binder, lower capacity retention than the in-situ polymerized PANi-SiNP composite electrode was obtained. Importantly, the uniform PANi coating on the Si particles also assists in enabling a deformable and stable SEI on the SiNP surface. We performed cell impedance measurements of the composite electrode after different cycles. As shown in Fig. 4a and Supplementary Fig. S3 , no obvious impedance increase was observed after cycles, indicating limited growth of the SEI during cycling. The impedance decrease for the first few cycles may be attributed to two major reasons: the slow wetting of electrolyte into porous battery electrodes, and the conductivity increase of SiNPs after lithium-ion doping associated with electrochemical charging. Indeed, as shown in Supplementary Fig. S3 , the impedance does not show obvious changes after cycling for more than 200 times. SEM images of composite electrodes after 2,000 electrochemical cycles confirmed that a uniform and thin SEI formed on the electrode, leading to the good cycling performance. 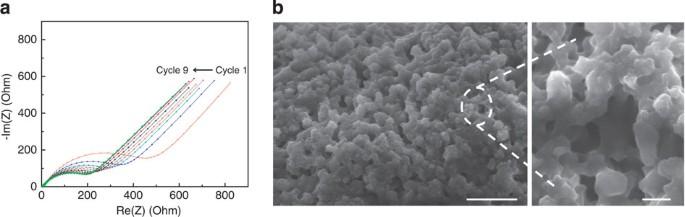Figure 4: Cell impedance test and characterization of SEI formation on composite electrodes. (a) Cell impedance tests of the SiNP-PANi composite electrode after each cycle between cycles 1 and 9. (b) SEM images of the electrode after 2,000 electrochemical cycles, showing that a uniform and thin SEI forms on the composite electrode. Scale bar, 1 μm (left) and 200 nm (right). Figure 4: Cell impedance test and characterization of SEI formation on composite electrodes. ( a ) Cell impedance tests of the SiNP-PANi composite electrode after each cycle between cycles 1 and 9. ( b ) SEM images of the electrode after 2,000 electrochemical cycles, showing that a uniform and thin SEI forms on the composite electrode. Scale bar, 1 μm (left) and 200 nm (right). Full size image In comparison, very thick SEI layers grow on SiNP electrodes with traditional PVDF binders ( Supplementary Fig. S4 ). The formation of a thin and stable SEI could potentially be attributed to the modification of the Si surface by the in-situ polymerization of PANi, similar to the polar hydrogen bonds between carboxyl groups of some binders and SiO 2 reported in recent studies [33] , [41] . Detailed investigation of this topic will be the subject of future studies. The stable SEI formation on our composite electrodes must be important for the long cycle life, as well as the high CE in the half-cell battery tests. In conclusion, we have developed a facile and scalable solution process to fabricate high-performance Li-ion battery negative electrodes by encapsulating SiNPs in a nanostructured 3D porous conductive polymer framework. By taking advantage of the conductive polymer matrix, which provides fast electronic and ionic transfer channels, as well as free space for Si volume changes, we successfully achieved high capacity and extremely stable electrochemical cycling. The electrode can be continuously deep cycled up to 5,000 times without significant capacity decay. Moreover, the solution synthesis and electrode fabrication process are highly scalable and compatible with existing slurry coating battery manufacturing technology. This will potentially allow for this high-performance composite electrode to be scaled up for manufacturing the next generation of high-energy Li-ion batteries, which are important for applications in electric vehicles and grid-scale energy storage systems that require both low-cost and reliable battery systems. In addition, our described materials design for silicon-based anodes may be extended to other battery electrode material systems that experience large volume changes and unstable SEI formation during cycling. Synthesis of electrode materials Composite SiNP-PANi hydrogel electrodes were made via the following solution processes. First, 0.9 ml solution A, which contains 100 mM aniline monomer and ~30 mM phytic acid, was added and mixed with 80 mg SiNPs (MTI, Inc.). Second, 0.3 ml solution B, containing 125 mM ammonium persulfate, was added into the above mixture and subjected to ~1 min bath sonication ( Supplementary Fig. S5 ). In about 2 min, the solution changed colour from brown to dark green and became viscous and gel-like, indicating in-situ polymerization of aniline monomer to form the PANi hydrogel. Electrode fabrication The SiNP/PANi electrode was made by doctor-blading the viscous SiNP-PANi hydrogel onto a Cu foil current collector (no binder used) and drying at room temperature. The SiNP-PANi hydrogel composite film was then mechanically pressed and thoroughly washed in deionized water several times to remove excess phytic acid, and the composite electrode film was dried in vacuum at room temperature for use in half cells as the working electrode. The total mass loading was typically 0.3–0.4 mg cm −2 . The Si mass loading is typically 0.2–0.3 mg cm −2 . We measured the yield of PAni in the reaction by obtaining the final weight of PAni hydrogel at the same recipe without the SiNP (after washing excessive monomers, acids and dried). With the yield value, we calculated the percent of Si in the composite to be 75%, or the Si to conductive hydrogel mass ratio of 3:1. The PANi hydrogel-only control samples were made via the same process by simply mixing the two solutions (solution A and solution B) without the addition of SiNPs. Cell assembly and electrochemical characterization The electrochemical properties were examined by galvanostatic cycling of coin-type half cells with the SiNP-PANi composite as the working electrode and lithium foil as the counter/reference electrode. The electrolyte for all tests was 1 M LiPF 6 in ethylene carbonate/diethylcarbonate/vinylene carbonate (1:1:0.02 v/v/v, Ferro Corporation), and separators (25 μm) from Asahi Kasei Co. were used. Calculation of volumetric capacity The thickness of the SiNP-PANi hybrid film was measured to be ~4.45 μm for an electrode with mass loading of 0.3 mg cm −2 . Therefore, the density ( ρ ) of the electrode is: The gravimetric capacity ( C g ) of our electrode is measured to be ~1,600 mAh g −1 as reported in Fig. 3 . The volumetric capacity ( C v ) is calculated: How to cite this article: Wu, H. et al . Stable Li-ion battery anodes by in-situ polymerization of conducting hydrogel to conformally coat silicon nanoparticles. Nat. Commun. 4:1943 doi: 10.1038/ncomms2941 (2013).